Comparative study of Co3O4(111), CoFe2O4(111), and Fe3O4(111) thin film electrocatalysts for the oxygen evolution reaction Water electrolysis to produce ‘green H 2 ’ with renewable energy is a promising option for the upcoming green economy. However, the slow and complex oxygen evolution reaction at the anode limits the efficiency. Co 3 O 4 with added iron is a capable catalyst for this reaction, but the role of iron is presently unclear. To investigate this topic, we compare epitaxial Co 3 O 4 (111), CoFe 2 O 4 (111), and Fe 3 O 4 (111) thin film model electrocatalysts, combining quasi in-situ preparation and characterization in ultra-high vacuum with electrochemistry experiments. The well-defined composition and structure of the thin epitaxial films permits the obtention of quantitatively comparable results. CoFe 2 O 4 (111) is found to be up to about four times more active than Co 3 O 4 (111) and about nine times more than Fe 3 O 4 (111), with the activity depending acutely on the Co/Fe concentration ratio. Under reaction conditions, all three oxides are covered by oxyhydroxide. For CoFe 2 O 4 (111), the oxyhydroxide’s Fe/Co concentration ratio is stabilized by partial iron dissolution. Recent years have seen a push towards renewable energy sources in the transition away from our dependence on fossil fuels. However, due to natural fluctuations of sources such as solar, wind, and tidal energy, an efficient energy storage path is needed for situations where the production level does not match the consumption. One potential route for energy storage is the electrocatalytic production of H 2 via water splitting. H 2 produced this way is called green hydrogen when the energy stems from renewable sources [1] , [2] . The limiting factor in this process is the sluggish kinetics of the oxygen evolution reaction (OER) and its high thermodynamic potential. Catalysts based on noble metals such as Ru and Ir exhibit excellent OER performance in acidic media, but their high cost conflicts with a large-scale use [3] . On the other hand, a number of oxides of less expensive, abundant metals have shown comparable reactivity in alkaline media, particularly oxide spinels containing Co, Ni, and Fe [2] , [4] . According to current knowledge, the real catalysts are not the oxides themselves, but surface oxyhydroxide layers which form under OER conditions [5] , [6] , [7] , [8] . Thus, the oxides are just pre-catalysts. Pure iron oxide was not predicted to yield a good catalyst [9] , but it was discovered that Fe-impurities in the electrolyte could enhance the activity of other oxides and oxyhydroxides [10] , [11] . This also holds for Co and Ni-based catalysts [12] , [13] , and it has been proposed that the active sites in iron-containing mixed oxyhydroxide catalysts are iron-based [14] , [15] , [16] . A recent study by Haase et al. reveals the presence of oxyl species on cobalt oxyhydroxide during OER, which may also play a relevant role for the reaction [17] . Understanding catalytic processes on nanoparticulate ‘real’ catalysts is demanding. For catalysis, the surface structure is relevant, but this can be very complex in such systems, and usually only incomplete knowledge is available. Moreover, the catalyst’s composition and structure are often inhomogeneous, which additionally enhances the complexity. Epitaxial thin film model catalysts are not afflicted by these issues: they have a well-defined surface structure and composition, and all parts of the surface can be equally well reached by the electrolyte. Furthermore, electrical conductivity, and its variation over the surface area can be a problem for the study of nanoparticulate ‘real’ catalysts, whereas homogeneous thin films with a thickness of just a few nanometres suffer much less from this issue even if the film material is nominally insulating. Consequently, results for epitaxial films can be more easily interpreted, and data for different films can be compared quantitatively if the experimental conditions are identical. Only very few experimental OER studies have been performed on well-ordered surfaces within the Co-Fe-O system. These include Co 3 O 4 (111) and CoOOH(001) [18] , [19] , [20] , CoO x nano-islands on Au(111) [21] , [22] , and Fe 3 O 4 (001) and (110) single crystal surfaces [23] , [24] . Building on the work of Bergmann et al. on polycrystalline Co 3 O 4 thin film catalysts [25] , Reikowski et al. elegantly showed that a thin layer of CoOOH is formed on the surface of Co 3 O 4 (111) in a rapid and reversible process that begins before the onset of OER [20] . Chung et al. recently reported that Fe ions in iron oxyhydroxides are “dynamically stable”, i.e., the ions are continuously dissolved from and redeposited onto the surface [26] . Müllner et al. used single crystal Fe 3 O 4 samples to show that the (001) and (110) surfaces are stable during OER, and that the (110) surface is more reactive [23] . Further, an operando study by Grumelli et al. demonstrated that the (√2×√2)R45° surface reconstruction of Fe 3 O 4 (001) is maintained deep into the OER regime and has a large effect on the OER kinetics [24] . Han et al. prepared Co x Fe 3-x O 4 films with different preferential orientations via electrodeposition on Cu single crystal substrates [27] and found that the OER activity depends on the surface orientation, with (110) > (111) > (001). The same orientation-reactivity trend was found by Poulain et al. for NiO thin films [6] . The central topic of the present study is the investigation of the effect of the Co/Fe concentration ratio on the OER activity for films of the same surface orientation [8] , [13] , [27] , [28] . We found the best OER reactivity and stability for mixed Co 1+δ Fe 2−δ O 4 (111) layers (|δ| <0.2) with a low Fe concentration, while pure cobalt oxide and iron oxide layers lag behind. However, Co 3 O 4 (111) freshly introduced into the electrolyte had an initial similar activity as the best Co 1+δ Fe 2 − δ O 4 (111) film, pointing towards a high activity of cobalt hydroxide which is unstable under OER conditions. Furthermore, for Co 1+δ Fe 2−δ O 4 (111), we observed a reduction of the Fe concentration by Fe dissolution into the electrolyte during OER, accompanied by an increase of the OER activity. Our results reveal that the cobalt/iron ratio is an important parameter for the OER reactivity of the films, while the surface morphology plays only a minor role. Pre- and post-electrochemistry characterization in ultra-high vacuum Well-defined epitaxial thin films were prepared via oxidative physical vapour deposition as discussed in the experimental section. The samples were characterized in situ with X-ray photoelectron spectroscopy (XPS), low-energy electron diffraction (LEED), and scanning tunnelling microscopy (STM) before and after the electrochemistry experiments. After more than 2 h under OER conditions, the oxide films still exhibited a visible LEED pattern, see Fig. 1 . The high background intensity after OER indicates a high level of surface disorder, most pronounced for Fe 3 O 4 (111). We assign this to remnants of the (oxy)hydroxide layers formed during OER [5] , [7] , [20] , [25] . They might be disordered and thus be partially responsible for the diffuse LEED background. The XPS data discussed later clearly reveal the presence of such layers. Fig. 1: LEED patterns of the thin films. Panels ( a – c ) before electrochemistry, ( d – f ) after electrochemistry. The electron energy was 160 eV. The  contrast of the images has been digitally enhanced to improve the visibility of the structures. Full size image The STM images in Fig. 2a–c show the general surface morphology of the as-prepared Co 3 O 4 (111), Fe 3 O 4 (111) and Co 1+δ Fe 2−δ O 4 (111) films. The step height of the terraces on all three films is ~4.8 Å, which is the distance between equivalent layers along [111]. The Fe 3 O 4 (111) film has terraces larger than 100 nm across, while the Co 1+δ Fe 2−δ O 4 (111) terraces are smaller, approximately 20–60 nm wide. Co 3 O 4 (111) exhibits an island-like structure, with terrace widths in the range of 10–30 nm. 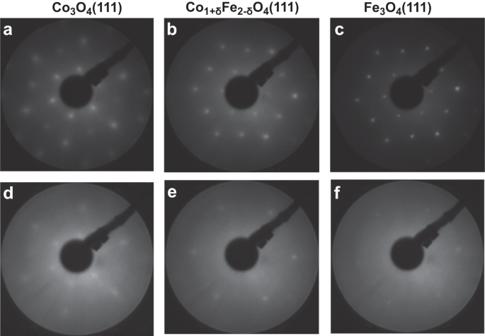Fig. 1: LEED patterns of the thin films. Panels (a–c) before electrochemistry, (d–f) after electrochemistry. The electron energy was 160 eV. The  contrast of the images has been digitally enhanced to improve the visibility of the structures. RMS roughness values are listed in Table 1 . The presence of steps and edges gives rise to an increased surface area, and therefore, the areas of the surface profiles are larger than the STM scan areas. The ratio of both (determined using the WSXM software [29] from several 500 × 500 nm STM images) is the scaling or roughness factor listed in Table 1 . By multiplying the area enclosed by the electrochemical cell (0.283 cm 2 ) by the scaling factor we can get an estimate of the electrochemically active surface area (ECSA) and find that the ECSA is not much different between the different as-prepared films. Fig. 2: STM images of the thin films. Panels ( a – c ) before, and ( d – f ) after more than 2 h of electrochemistry. Tunnelling conditions: ( a – c , e , f ) sample bias 2.0 V, current 0.1 nA, ( d ) 3.0 V, 0.2 nA. Full size image Table 1 Root mean square (RMS) roughness, surface area scaling factor, electrochemical surface area (ECSA), and specific capacitance, C s , for Co 3 O 4 (111), Co 1+δ Fe 2−δ O 4 (111), and Fe 3 O 4 (111) before and after OER (oxygen evolution reaction) Full size table In order to determine the specific capacitance, C s [30] , we divided the double-layer capacitance measured with potentiostatic electrochemical impedance spectroscopy (PEIS) (Supplementary Fig. S1 and Supplementary Table S1 ) by the ECSA listed in Table 1 . Interestingly, the values of C s for the Co 3 O 4 (111) surface are ~3 times larger than those determined for metallic Co [30] , which may be due to different surface structures and oxidation states. An investigation of the Co 1+δ Fe 2−δ O 4 (111) surface structure has not yet been reported. Quantitative XPS analysis finds an enhanced iron concentration in the surface-sensitive spectra for as-prepared Co 1+δ Fe 2−δ O 4 (111) (see Supplementary Fig. S2 ), indicating that the terminating layer consists mostly of iron. In agreement with that, atomic resolution STM images (panels d,e of Supplementary Fig. S3 ) exhibit similar arrangements of protrusions for Fe 3 O 4 (111) and Co 1+δ Fe 2−δ O 4 (111). Thus, the combined information from STM, LEED, and XPS infers that tetrahedrally terminated Fe 3 O 4 (111) terminates most of the Co 1+δ Fe 2−δ O 4 (111) surface (Supplementary Fig. S4 ). This is plausible, since Co 3 O 4 (111) and Fe 3 O 4 (111) are both terminated by tetrahedral layers [31] , [32] , [33] , and Co 1+δ Fe 2−δ O 4 (111) might share this termination, being a mixture of both. Comparison of the Fe 3 O 4 (111) and Co 1+δ Fe 2−δ O 4 (111) STM images recorded before and after electrochemistry (Fig. 2 ) reveals that the terrace structures are not significantly modified, as also reflected in the small changes in the RMS roughness (see Table 1 ). The latter gets slightly smaller, indicating that the OER remnants tend to smoothen the surface by filling the valleys. On the other hand, the Co 3 O 4 (111) surface is more granular after electrochemistry: the density of islands has approximately doubled, and the RMS roughness is ~40% larger (Table 1 ). After electrochemistry, there is clearly an enhanced short-scale roughness for Fe 3 O 4 (111) on the terraces, accompanied by a notable surface area increase and a C s decrease. This may be related to the oxidation of the film (see discussion below) or structural rearrangements during the formation of the oxyhydroxide layer. O 1 s and metal 2 p XPS spectra are compiled in Fig. 3 . The O 1 s spectra of all three films (panels a-c) show the main oxide peak at ~530 eV and after electrochemistry an additional small peak at about 1.5 eV higher binding energy, which we assign to surface hydroxide. Oxyhydroxide O1 s peaks overlap with the oxide bulk peak and are therefore not clearly detectable [34] . Yang et al. identified the cobalt hydroxide O 1 s bulk peak at 531.2 eV, somewhere between the surface hydroxide and the bulk oxide peak [35] , which makes it hard to clearly identify it. Since the layer may also contain oxyhydroxide, we use the notation ‘(oxy)hydroxide’ when we refer to the full layer. Assuming a flat and homogeneous layer, we find a surface (oxy)hydroxide layer thickness in the range of 3 Å for all three oxides. The whole surface layer may not be much thicker, as concluded from the intensity of the LEED spots after OER (see Fig. 1 ), which would be compatible with a flat layer less than ~1 nm thick (for details see SI). For Fe 3 O 4 (111) it was checked whether the hydroxide stems from the electrochemical experiments by recording an O 1 s spectrum from a sample area not exposed to the electrolyte (Supplementary Fig. S5 ). The much weaker hydroxide-related O 1 s intensity shows that the hydroxide layer indeed results mostly from the OER electrochemistry. It is expected that the same holds for the Co 3 O 4 (111) and Co 1+δ Fe 2−δ O 4 (111) samples. Fig. 3: X-ray photoelectron spectroscopy (XPS) spectra from the O 1 s and metal 2p regions recorded before (blue lines) and after (red lines) electrochemistry (offset for clarity). Panels ( a , d ): Co 3 O 4 (111), ( b , e , f ): Co 1+δ Fe 2−δ O 4 (111), ( c , g ): Fe 3 O 4 (111). Difference spectra (‘After’–‘Before’) are plotted using olive lines. Peak fits for the O 1s spectra after electrochemistry are shown as thin red and brown lines. Prior to the calculation of the 2 p difference spectra, the 2 p spectra recorded before electrochemistry were shifted on the energy axis (to compensate for band bending effects) to align them with the spectra recorded after electrochemistry and they were normalized to identical peak areas to reveal changes of the electronic structure. Therefore, concentration changes are masked in the different data. Full size image Contaminants were absent according to the XPS spectra, except for a minute amount of adventitious carbon (<1 monolayer). Substrate material (Pt or Au) could not be detected (Supplementary Fig. S6 ), indicating that all films are closed. The Fe 2 p spectra of the pure Fe 3 O 4 (111) film, Fig. 3g , reveal a strongly reduced Fe 2+ intensity after OER. This will (in part) be due to oxyhydroxide formed during OER, but in view of the limited thickness of the layer, one may expect that also part of the oxide becomes oxidized to Fe 2 O 3 . Such an oxidation process has also been observed for Fe 3 O 4 (100) by Müllner et al. [23] . and for Fe 3 O 4 nanocubes by Hsu et al. [36] . The Fe 3 O 4 (111) LEED pattern of the oxide after OER shows spots at similar positions as before OER, see Fig. 1c, f , which would be compatible with the formation of maghemite (γ-Fe 2 O 3 ), which is cubic and can be formed by dissolution of tetrahedrally-coordinated iron out of the Fe 3 O 4 lattice leading to a Fe oxidation state of 3+ without changing the lattice structure. As shown in Table 1 , the specific capacitance of the Fe 3 O 4 (111) film has decreased by ~25 %, which we attribute to the oxidation process. For Co 3 O 4 (111), the Co 2 p spectrum (panel d) is very similar to spectra reported by others [37] and is not affected very much by the OER process, which means that the oxide is mostly stable under the chosen OER conditions. The features in the difference spectrum at around 780 eV are consistent with the formation of CoOOH at the surface [37] , [38] . Likewise, the small shift of the main lines to slightly higher binding energy would be compatible with the formation of CoOOH and Co(OH) 2 [35] . For the Co 1+δ Fe 2−δ O 4 (111) film, the Co 2 p spectra recorded before and after electrochemistry (panel e) are also very similar, with very small CoOOH-related features in the region around 780 eV. 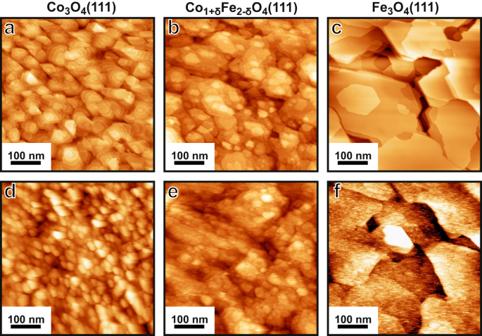Fig. 2: STM images of the thin films. Panels (a–c) before, and (d–f) after more than 2 h of electrochemistry. Tunnelling conditions: (a–c,e,f) sample bias 2.0 V, current 0.1 nA, (d) 3.0 V, 0.2 nA. Within the composition range |δ| <=0.2, the spectra do not vary much and therefore only data for a selected film (Film 1, Table 2 ) are shown. Clearly, the Co 2 p spectrum of Co 1+δ Fe 2−δ O 4 (111) is different from the corresponding Co 3 O 4 (111) spectrum in panel d, which results from the fact that the cobalt ions in Co 1+δ Fe 2−δ O 4 (111) are in a 2+ oxidation state, and therefore, the Co 2 p spectrum is similar to that of CoO [37] . Table 2 Fe concentrations (the cobalt concentration is C Co = 100-C Fe ) as a percentage of the total metal content for the prepared Co 1+δ Fe 2−δ O 4 (111) films before and after oxygen evolution reaction (OER) experiments Full size table A quantitative evaluation of the Co 2 p and Fe 2 p spectra of the Co 1+δ Fe 2−δ O 4 (111) films reveals a decrease of the Fe concentration during electrochemistry in all experiments. Table 2 shows that the decrease is more pronounced in the surface-sensitive spectra, which demonstrates that the iron loss occurs at the surface. No significant changes of the Co 1+δ Fe 2−δ O 4 (111) surface compositions were observed when the samples were placed in the electrolyte without applied potential, which shows that the iron loss only occurs under OER conditions (see Supplementary Fig. S7 ). An OER run performed for 10 min instead of 2 h showed a similar loss, indicating that it occurred mostly within the first 10 min. However, there are probably also some long-term losses as indicated by Supplementary Fig. S8 , which reveals an activity improvement for more than 20 h. The Fe 2+ intensity of Co 1+δ Fe 2−δ O 4 (111) is reduced after OER, revealing that part of the surface iron is oxidized. Oxyhydroxide formation and oxidation of the iron oxide at the surface may be responsible for this. The Co 2+ ions are apparently not further oxidized under the given OER conditions, similar to the observation for Co 3 O 4 (111). Electrochemical measurements Cyclic voltammetry (CV) was applied to identify the influence of Fe on the surface redox electrochemistry. Before a 2-h OER run, linear sweep voltammograms (LSVs) were recorded from the open-circuit voltage (OCV) up to OER conditions (defined here as the potential where the current density reaches 1 mA/cm 2 ), see Fig. 4a, b . Fig. 4: Cyclic voltammograms of Co 3 O 4 (111), Fe 3 O 4 (111), and Co 1+δ Fe 2−δ O 4 (111) thin films. The data in ( a , b ) were recorded at the beginning of the experiment from the open-circuit voltage (OCV) up to 1 mA/cm 2 , and the data in ( c , d ) after 2 h at OER (oxygen evolution reaction) conditions starting with a cathodic sweep. Panels ( a ) and ( c ) show the redox transition region. In ( a ) the second anodic sweep of the Fe 3 O 4 (111) sample is displayed to show the disappearance of the redox transition at ~1.26 V. Scan rate: 5 mV/s. Electrolyte: 0.1 M KOH. Cathodic scans are shown as dashed lines. The arrow in panel ( b ) marks the potentials where the current densities reach 1 mA/cm 2 . These potentials were employed for the subsequent CA measurements. For Co 1+δ Fe 2−δ O 4 (111), data from the film with the lowest Fe concentration are shown [Film 1, Table 2 ]. The resistances for the IR correction and the high-frequency cell resistances are listed in Supplementary Tables S2 and S3 , respectively. Full size image For the Co 3 O 4 (111) film, a redox feature is visible at ~1.46 V. This feature has typically been assigned to a Co 3+ /Co 4+ redox transition [39] , [40] . The assignment is likely a strong simplification as it neglects metal-ligand charge reorganization leading to electron–hole formation at surface oxygen ions, similar to IrO x [17] , [41] . There is no indication of a peak previously reported between 1.0 and 1.3 V for other Co-based electrocatalysts [18] , [25] , [42] . We note that a peak at this potential has been observed more frequently for layered CoOOH-like structures than for Co 3 O 4 -like oxides [25] . The first anodic linear sweep of the Fe 3 O 4 (111) film exhibits broad oxidation features centred at approximately 0.73 V (Supplementary Fig. S9 ) and 1.26 V vs RHE. These features only appear in the first sweep, and no reduction is observed during the following cathodic scan, nor further oxidation on later anodic sweeps up to OER conditions. We tentatively assign these transitions to the oxidation of near-surface iron atoms in the context of the Fe 3 O 4 → Fe 2 O 3 transformation. These redox features were completely missing in the Fe 3 O 4 (001) CV data published by Grumelli et al. [24] . However, Calvillo et al. observed peaks at ~1.25 V during the first two CVs for Fe 3 O 4 /Pd(001) films [43] . 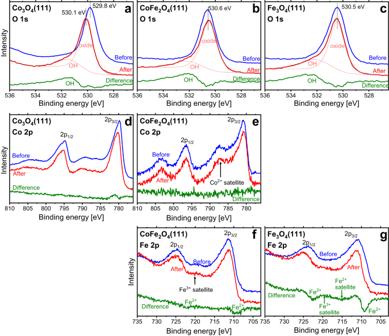Fig. 3: X-ray photoelectron spectroscopy (XPS) spectra from the O 1sand metal 2p regions recorded before (blue lines) and after (red lines) electrochemistry (offset for clarity). Panels (a,d): Co3O4(111), (b,e,f): Co1+δFe2−δO4(111), (c,g): Fe3O4(111). Difference spectra (‘After’–‘Before’) are plotted using olive lines. Peak fits for the O 1s spectra after electrochemistry are shown as thin red and brown lines. Prior to the calculation of the 2pdifference spectra, the 2pspectra recorded before electrochemistry were shifted on the energy axis (to compensate for band bending effects) to align them with the spectra recorded after electrochemistry and they were normalized to identical peak areas to reveal changes of the electronic structure. Therefore, concentration changes are masked in the different data. An approximately linear offset is seen in the initial Fe 3 O 4 (111) CVs (see Supplementary Fig. S9 ). The background current observed may be due to a slow oxidation process in the bulk of the film. In the CVs obtained after OER this background is not present anymore, which is another indication that it is related to the Fe 3 O 4 → Fe 2 O 3 transformation, since the oxidation process may be largely complete or have slowed down after OER. The initial anodic scan of the Co 1+δ Fe 2−δ O 4 (111) films had no distinguishable redox features. This may be because the Fe in Co 1+δ Fe 2−δ O 4 is already in a 3+ oxidation state [44] , which is probably also the case for most of the surface iron atoms (there is only a small Fe 2+ contribution, see Fig. 3f ). As discussed, the cobalt concentration at the surface of the pristine sample is probably small, which could explain why Co redox transitions were not detected. 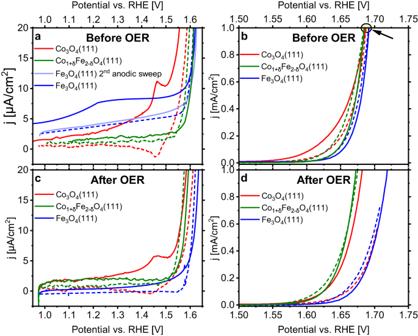Fig. 4: Cyclic voltammograms of Co3O4(111), Fe3O4(111), and Co1+δFe2−δO4(111) thin films. The data in (a,b) were recorded at the beginning of the experiment from the open-circuit voltage (OCV) up to 1 mA/cm2, and the data in (c,d) after 2 h at OER (oxygen evolution reaction) conditions starting with a cathodic sweep. Panels (a) and (c) show the redox transition region. In (a) the second anodic sweep of the Fe3O4(111) sample is displayed to show the disappearance of the redox transition at ~1.26 V. Scan rate: 5 mV/s. Electrolyte: 0.1 M KOH. Cathodic scans are shown as dashed lines. The arrow in panel (b) marks the potentials where the current densities reach 1 mA/cm2. These potentials were employed for the subsequent CA measurements. For Co1+δFe2−δO4(111), data from the film with the lowest Fe concentration are shown [Film 1, Table2]. The resistances for the IR correction and the high-frequency cell resistances are listed in Supplementary TablesS2andS3, respectively. The peak expected between 1.0 and 1.3 V RHE may be absent for a similar reason as discussed for Co 3 O 4 (111). Additionally, the presence of Fe has been shown to shift the Co oxidation peaks to higher potentials [28] . Therefore, the peak that we observe at 1.46 V for Co 3 O 4 (111) may be obscured by the onset of OER if it does exist for Co 1+δ Fe 2−δ O 4 (111). After the initial CVs, the samples were exposed to OER conditions for 2 h using the potential where the current density reached 1 mA/cm 2 in the preceding CV scan (see arrow mark in Fig. 4b ). During the 2-h period at OER conditions, chronoamperometry (CA) data were recorded to reveal the time dependence of the current, see Supplementary Fig. S10 . Following OER, further CVs were measured, which are shown in Fig. 4c , d. These data reveal that the onset of the Fe 3 O 4 (111) activity after OER is at a significantly higher potential than before OER. Co 3 O 4 (111) has a similar onset potential to Fe 3 O 4 (111) in the cathodic scan after OER, but is much better in the subsequent anodic scan, while the Co 1+δ Fe 2−δ O 4 (111) film has a lower onset potential after OER. OER activity data for a potential of 1.63 V RHE are compiled in Fig. 5 for the thin film oxides using data from linear sweep voltammograms measured at various stages of the experiment. We note that the OER activity was calculated taking into account the surface roughness and thus, correspond to the intrinsic activity of the exposed surfaces. The experimental first step was a CV cycle (an anodic LSV from open circuit potential to OER potential, followed by a cathodic LSV to 1 V RHE ). Following this, the potential was brought back to that for j = 1 mA/cm 2 and held for at least 2 h. Then, a further CV scan was performed (a cathodic LSV from the potential applied during OER down to 1 V RHE , followed by an anodic sweep back to OER conditions). 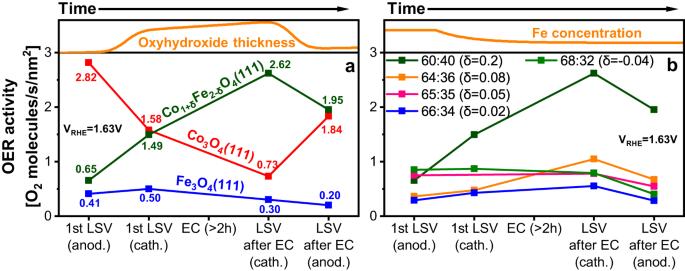Fig. 5: Oxygen evolution activies of the thin films at different stages of the experiment. Panels (a) Co3O4(111), Co1+δFe2−δO4(111), and Fe3O4(111) thin films,  (b) Co1+δFe2−δO4(111) thin films with differing Fe:Co ratios. Data for the Co1+δFe2−δO4(111) film with the lowest Fe concentration (δ = 0.2) are shown in (a). The oxyhydroxide layer thickness plot in the top panel in (a) and the Fe concentration plot in the top panel in (b) are qualitative guesses based on a report that the oxyhydroxide layer thickness increases with increasing potential20and the observation of a decreasing Fe concentration during OER in this study, respectively. ‘anod.’ means ‘anodic’ and ‘cath.’ means ‘cathodic’, both describing the scan direction. The activities are given as the number of O2molecules per second and square nanometre for VRHE= 1.63 V. Figure 5 displays the activities derived from the current densities at V RHE = 1.63 V during the first CV and the CV after 2 h at OER conditions. Thus, Fig. 5 illustrates condition- and time-dependent trends in the activity of the catalysts. The activity data can be quantitatively compared among the thin films, since the electrochemistry experiments were performed under identical conditions and the ECSAs are well known, see Table 1 . Since the data shown at the third abscissa point in Fig. 5 , ‘LSV after EC (cathodic)’ were obtained directly after the extended OER scan, they are likely the best representation of the activities of the catalysts under reaction conditions. In panel a, Co 1+δ Fe 2−δ O 4 (111) (δ = 0.2) was the most active catalyst at this point. We also found a clear trend in the dependence of the activity on the Fe concentration in Co 1+δ Fe 2−δ O 4 (111) in the given concentration range: films with a lower Fe concentration have the higher activity, see panel b. The dependence is significant—the activity varies by several times with a change in Fe concentration of only a few percent. Fig. 5: Oxygen evolution activies of the thin films at different stages of the experiment. Panels ( a ) Co 3 O 4 (111), Co 1+δ Fe 2−δ O 4 (111), and Fe 3 O 4 (111) thin films,  ( b ) Co 1+δ Fe 2−δ O 4 (111) thin films with differing Fe:Co ratios. Data for the Co 1+δ Fe 2−δ O 4 (111) film with the lowest Fe concentration (δ = 0.2) are shown in ( a ). The oxyhydroxide layer thickness plot in the top panel in ( a ) and the Fe concentration plot in the top panel in ( b ) are qualitative guesses based on a report that the oxyhydroxide layer thickness increases with increasing potential [20] and the observation of a decreasing Fe concentration during OER in this study, respectively. ‘anod.’ means ‘anodic’ and ‘cath.’ means ‘cathodic’, both describing the scan direction. The activities are given as the number of O 2 molecules per second and square nanometre for V RHE = 1.63 V. Full size image Under OER conditions, the iron oxide film is covered by an FeOOH layer [7] , which is soluble in basic media, and dissolves slowly during OER, with the rate of dissolution depending on the potential applied [45] . At high anodic potentials it is rapidly oxidized to FeO 4 2− , which is highly reactive but also highly soluble [45] . An ICP-MS (inductively coupled plasma mass-spectrometry) characterization of the iron content in the electrolyte revealed a slight increase after electrochemistry, which corresponds to the dissolution of just 0.4 nm of Fe 3 O 4 . This is a negligible part of the Fe 3 O 4 (111) film, which had a thickness between 10 and 15 nm. The data in Fig. 5 also revealed that the activity of Fe 3 O 4 (111) is the lowest of the three catalysts. After a brief improvement at the beginning, it degrades until it finally reaches about 50% of the starting activity. This degradation may in part be due to the oxidation towards Fe 2 O 3 , which is an electrical insulator, but the fact that the activity is the smallest at all abscissa points in Fig. 5 suggests that the oxyhydroxide layer on Fe 3 O 4 (111) simply has a low OER activity, as also proposed by other authors [9] . To obtain insights into the state of the thin films during OER, operando Raman spectra were recorded. The spectra support the XPS result that part of the film transforms to γ-Fe 2 O 3 during OER (Supplementary Fig. S11 and accompanying discussion). No (oxy)hydroxide-related peaks could be found in any of the Raman spectra even after extended times (>1 h) under OER conditions. This indicates that the oxyhydroxide film was too thin for a detectable signal. Operando X-ray scattering was also applied, but also here, the oxyhydroxide could not be clearly detected. This is in line with the results of Wiegmann et al. [46] . who found that the oxyhydroxide layer formed on an Co 3 O 4 (111) layer grown in ultra-high vacuum (UHV) is very thin, thinner than on electrochemically grown Co 3 O 4 (111) layers. It may be assumed that structural imperfections in the latter give rise to this difference. Figure 5a suggests that the formation and conditioning of the oxyhydroxide layer on Co 3 O 4 (111) has a detrimental effect on the activity: before electrochemistry, the Co 3 O 4 (111) activity is higher than that of the other oxides, but the activity decreases once OER conditions have been reached and it keeps decreasing with increasing OER time. This is also visible in Supplementary Fig. S10 , which shows that the Co 3 O 4 (111) OER current density decreases continuously after the start of the experiment. During the cathodic scan after the EC experiments, the activity is as small as that of Fe 3 O 4 (111) while the Co 3 O 4 (111) OER activity improves again when the potential is decreased and the film exposed to reducing conditions, see the last data point in Fig. 5a . One possible conclusion from this observation is that the activity of the surface layer, probably mostly hydroxide, which forms after exposure of the sample to the electrolyte [47] is higher than that of the thermodynamically more stable oxyhydroxide layer which forms under OER reaction conditions. An oxyhydroxide layer with an initially high iron concentration may form on Co 1+δ Fe 2−δ O 4 (111) due to oxide’s high surface iron concentration, which may be the reason for the similar activities of Fe 3 O 4 (111) and Co 1+δ Fe 2−δ O 4 (111) in the initial phase of the experiment, Fig. 5 , and also for the similar slopes of the Fe 3 O 4 (111) and Co 1+δ Fe 2−δ O 4 (111) CA curves in the first ~50 s, see Supplementary Fig. S10 . Beyond this time, the Fe 3 O 4 (111) and Co 1+δ Fe 2−δ O 4 (111) CA curves deviate more and more with increasing time. Burke et al. found that (Co,Fe)OOH mixed oxyhydroxide electrodes dissolve in a KOH electrolyte during OER when the Fe concentration is larger than 54%, but they are stable at lower Fe concentrations [28] . We find a reduction of the surface Fe concentration to similar values, see Table 2 for Co 1+δ Fe 2−δ O 4 (111) after OER. An ICP-MS characterization of the electrolyte after OER showed the same Fe loss as for the Fe 3 O 4 (111) film (i.e., ~0.4 nm), but no increase of the Co concentration in the electrolyte, indicating that Co is not lost from the film. We hypothesize that iron dissolves into the electrolyte from the oxyhydroxide layer without re-deposition. To test this hypothesis, a Co 1+δ Fe 2−δ O 4 (111) film was prepared, but in the final preparation step, pure Fe was deposited instead of a Fe/Co mixture. After oxidizing the film, the excess Fe was still not well-mixed within the film, and it remained as an Fe 3 O 4 (111)-like layer on the surface. A long-term OER CA scan (~21 h, see Supplementary Fig. S8 ) revealed that for about 1 h the film behaved similar to Fe 3 O 4 (111), where the current mostly decreases as a function of time, see Supplementary Fig. S10 . However, after this the current increased, which we attribute to iron dissolution and the concomitant enrichment of cobalt in the oxyhydroxide layer. The Fe concentration following the CA scan was ~50%. Details are discussed in the SI (Supplementary Fig. S8 ). Summing up, we have performed a comparative study of the OER activity of epitaxial crystalline thin oxide film model catalysts: Co 3 O 4 (111), Co 1+δ Fe 2−δ O 4 (111) (|δ| <=0.2), and Fe 3 O 4 (111). Epitaxial, well-characterized and defect-poor UHV-grown cobalt ferrite layers are used here for the first time for OER studies and permit to quantitatively assess the effect of the iron concentration on the reactivity, which may be a topic for future studies. Co 3 O 4 (111) and Co 1+δ Fe 2−δ O 4 (111) were largely stable under the chosen OER conditions, but Fe 3 O 4 (111) was found to partially transform to the cubic γ-Fe 2 O 3 phase. Co 1+δ Fe 2−δ O 4 (111), the most active catalyst, was found to lose iron during OER via dissolution, eventually converging towards a stable low Fe concentration, while cobalt dissolution was not detected. The Co 3 O 4 (111) surface appears to be somewhat granular after 2 h of OER, while the surface island structures of Co 1+δ Fe 2−δ O 4 (111) and Fe 3 O 4 (111) remained nearly unchanged. Co 3 O 4 (111) has an initial high OER activity which decreases when the OER reaction is running, which we attribute to a higher activity of the surface layer formed after introduction into the electrolyte comprising a higher density of reduced Co 2+ sites and hydroxyls. In contrast, the Co 1+δ Fe 2−δ O 4 (111) activity increases during exposure to OER conditions and decreases upon exposure to reducing conditions. We attribute this finding to the compositional adaptations leading to elevated Fe surface concentration passivating the surface. We feel that the most important aspect of the thin-epitaxial-film approach is a significant reduction of uncertainties inherent to less well-defined pre-catalyst systems, which permits quantitative comparison of the specific activity for different oxides. Given the homogeneity of the surfaces, we can use laterally averaging spectroscopy methods without averaging over differing areas. These data will constitute a feedstock for theoretical modelling which is likely needed to further unravel mechanistic details of the reaction process but also require more advanced surface sensitive chemical spectroscopy. Upcoming studies will also involve the effect of the facet terminating the surface and thereby, provide further needed insights to yield in a comprehensive picture of the oxygen evolution surface of Co-based electrocatalysts for alkaline water splitting. Experimental chamber An UHV chamber with a base pressure of 4 × 10 −11 mbar was used for sample preparation and surface characterization with XPS, LEED, and STM at room temperature. For some measurements the surface sensitivity of XPS was enhanced by measuring at non-normal detection angles. Unless stated otherwise, measurements were made at normal emission geometry (0°) using Mg Kα radiation (1253.6 eV). Further details of the UHV chamber may be found in the supporting information. Thin film preparation We have developed recipes for the production of well-ordered epitaxial thin films of Co 1+δ Fe 2−δ O 4 (111) on Pt(111) and Co 3 O 4 (111) on Au(111). A well-established preparation procedure was employed for Fe 3 O 4 (111) films on Pt(111) [48] . All samples were prepared and characterized quasi in situ in UHV before and after OER without exposure to air at any point to avoid surface contaminations. ‘Quasi in-situ’ means here that all experimental steps were done in the same system, but in different interconnected chambers and environments (UHV, liquid, 1 bar Ar), without intermediate exposure to air during the sample transfer. The Pt(111) and Au(111) crystal substrates (MaTeck GmbH, Germany) were prepared through cycles of Ar + -sputtering and annealing in UHV until a sharp LEED pattern with a low background intensity was observed and no traces of carbon were detected with XPS. Fe and Co were deposited using e-beam assisted evaporators (EFM 4, Omicron) with the deposition rates being calibrated with a quartz microbalance. Deposition rates of 1.2 Å/min for Fe and 0.6 Å/min for Co were employed, except for the growth of Co 3 O 4 (111), where a Co deposition rate of 1.3 Å/min was used. The Fe 3 O 4 (111) film was grown on a Pt(111) substrate by molecular beam epitaxy (MBE) using a slightly modified version of the procedure described by Sala et al. [48] . First, 4.1 Å of Fe was deposited at room temperature. The sample was then heated in 1 × 10 −6 mbar O 2 from room temperature up to 1000 K, where it was held for 2 min. The O 2 pressure was not reduced until the sample had cooled down to 500 K after annealing. This led to the formation of an FeO(111) layer covering the whole substrate. Then, in at least 3 cycles, ~20 Å of Fe were deposited at room temperature followed by annealing in 5 × 10 −6 mbar of O 2 for 20 min. This led to films approximately 10–15 nm thick. The oxidation temperature was limited to 850 K to avoid de-wetting of the film. This limited temperature resulted in broader LEED spots and smaller terraces, but partial exposure of the Pt substrate could have led to misleading electrochemical data and therefore had to be avoided. A recipe for the preparation of Co 3 O 4 (111) on Ir(100) films has been published [32] , but in view of the high OER activity of Ir we decided to avoid this metal as underlayer and developed a new procedure to prepare Co 3 O 4 (111) on Au(111). First, a buffer layer of 2.4 nm of Co was deposited at ~250 K. Following this, 1.6 nm of Co was deposited in 5 × 10 −6 mbar O 2 at ~350 K. While maintaining this O 2 pressure, the sample was heated to 650 K and kept at this temperature while 1.9 nm of Co was deposited. After this, the sample was annealed at 650 K for 10 min. The valve allowing O 2 into the chamber was closed when the annealing was stopped. The thickness of these films was approximately 10–12 nm. Co 1+δ Fe 2−δ O 4 (111) films were prepared on Pt(111) by following a procedure similar to that used for growing Fe 3 O 4 (111) films on Pt(111) [49] . First, an FeO layer was prepared as detailed above. Following this, Fe and Co were simultaneously deposited at room temperature for ~18 min, followed by annealing in 1 × 10 −5 mbar O 2 for at least 30 min at 850 K. This deposition and oxidation cycle was repeated at least three times. Annealing temperatures were limited to 850 K, as for Fe 3 O 4 (111). The stoichiometry of the layers was judged from Fe 2 p and Co 2 p XPS spectra. If required, it was adjusted by the addition of iron or cobalt combined with annealing and oxidation. The small differences in the final concentrations of iron and cobalt within these films, denoted Co 1+δ Fe 2−δ O 4 (111), did not lead to large differences in the LEED and STM data. These films were 15–20 nm thick. Some STM images and LEED patterns of as-prepared Co 3 O 4 (111), Co 1+δ Fe 2−δ O 4 (111), and Fe 3 O 4 (111) are shown in Supplementary Fig. S3 . According to published studies [31] , [50] the Fe 3 O 4 (111) surface is terminated with a layer of iron atoms under UHV conditions. In the bulk, these iron ions would be in tetrahedral positions. At the surface, the Co–O coordination in Co 3 O 4 (111) is unsaturated (lower than 4-fold), but the layer is still commonly called ‘tetrahedral’. Based on an IV-LEED study of Co 3 O 4 (111)/Ir(100) [33] , Co 3 O 4 (111) is terminated with a ‘tetrahedral’ Co layer. Electrochemical tests We investigated the electrochemical (EC) performance of the thin films in an electrochemical cell attached to the UHV chamber, allowing transfer in situ without exposure to air. Details of the electrochemistry setup can be found in Supplementary Fig. S12 and discussion. Following electrochemistry, the sample was rinsed using ultrapure water before being reintroduced to the load-lock chamber. The load lock was pumped down to UHV using a turbomolecular pump, before the sample was reintroduced to the UHV analysis chamber for post-electrochemistry analysis. The following protocol was used for the electrochemical measurements. First, the electrolyte was introduced with the sample at OCV. Then, at OCV + 0.04 V, PEIS was measured, followed by cyclic voltammograms (CVs). The first anodic sweep was from the previous potential, slightly above OCV, to the potential where the current density reached 1 mA/cm 2 . The following CV cycle was between 1 V RHE and the potential corresponding to 1 mA/cm 2 . Then a PEIS spectrum was recorded with the potential at this value. The measured resistance was used for iR correction. Following this, chronoamperometry (CA) data were recorded with the sample at the same potential for approximately 2 h to observe time-dependent reactivity changes. Then, another CV was measured: the first LSV was cathodic, starting from the potential applied during OER down to 1 V RHE , followed by an anodic scan to the potential where the current density reached 1 mA/cm 2 . After this, a PEIS spectrum was measured at OER conditions (1 mA/cm 2 ). Finally, the seal between the sample and the cell was removed while this potential was still being applied. This was to ensure that the sample did not return to OCV in the electrolyte, as this might induce additional changes at the surface, which might affect the post-reaction surface characterization results. All given potentials and all potential scales are iR-corrected and referenced to the reversible hydrogen electrode (RHE). In all the electrochemical experiments, we used 0.1 M KOH and calibrated the Ag/AgCl reference electrode against a commercial RHE in the same electrolyte to compensate for any deviations from the nominal pH. For the reference electrode calibration, we measured the open circuit potential between the Ag/AgCl reference electrode and the RHE in the electrolyte after equilibration for at least 15 min. [We note that a potentially wrong calibration of the reference electrode might cause stronger deviations in the current compared to the variations in the OH- concentrations due to errors in the weighting of the chemicals.] We did not specify the pH of the electrolyte in the manuscript to avoid any misleading or wrong statements. The ohmic resistance of the electrochemical setup was determined from a Nyquist plot obtained via potentiostatic impedance spectroscopy as the high-frequency resistance HFR (HFR = Re(Z) at Im(Z) = 0 Ω). Operando Raman measurements Operando Raman measurements were conducted using a Renishaw (InVia Reflex) confocal Raman microscope. The electrochemical measurements were performed in a 0.1 M KOH electrolyte in a home-built spectro-electrochemical cell made of Teflon and controlled by a Biologic SP240 potentiostat. The cell was equipped with a reference electrode (leak-free Ag/AgCl, Alvatek) and a counter electrode (Pt foil). The substrate crystal with the thin film was fixed in place using Kapton tape. The sample was transferred from the UHV chamber to the cell through air. Further details of the operando Raman measurements may be found in the SI.